Full-length TDP-43 forms toxic amyloid oligomers that are present in frontotemporal lobar dementia-TDP patients Proteinaceous inclusions are common hallmarks of many neurodegenerative diseases. TDP-43 proteinopathies, consisting of several neurodegenerative diseases, including frontotemporal lobar dementia (FTLD) and amyotrophic lateral sclerosis (ALS), are characterized by inclusion bodies formed by polyubiquitinated and hyperphosphorylated full-length and truncated TDP-43. The structural properties of TDP-43 aggregates and their relationship to pathogenesis are still ambiguous. Here we demonstrate that the recombinant full-length human TDP-43 forms structurally stable, spherical oligomers that share common epitopes with an anti-amyloid oligomer-specific antibody. The TDP-43 oligomers are stable, have exposed hydrophobic surfaces, exhibit reduced DNA binding capability and are neurotoxic in vitro and in vivo . Moreover, TDP-43 oligomers are capable of cross-seeding Alzheimer’s amyloid-β to form amyloid oligomers, demonstrating interconvertibility between the amyloid species. Such oligomers are present in the forebrain of transgenic TDP-43 mice and FTLD-TDP patients. Our results suggest that aside from filamentous aggregates, TDP-43 oligomers may play a role in TDP-43 pathogenesis. Inclusion bodies (IBs) of the transactive response DNA-binding protein 43 (TDP-43) are pathologic hallmarks of frontotemporal lobar degeneration with τ- and α-synuclein-negative but ubiquitin-positive inclusions (previously designated as frontotemporal lobar dementia (FTLD)-U, and recently known as FTLD-TDP) and amyotrophic lateral sclerosis (ALS) [1] , [2] , [3] . FTLD-TDP is one of the major subtypes of FTLD [4] and the second most prevalent cortical dementia occurring before the age of 65 years [5] . ALS is a neurodegenerative disease characterized by relentless loss of motor neurons followed by progressive weakness and muscular wasting, which results in paralysis and death. FTLD-TDP and ALS, together with several other neurodegenerative diseases, are categorized as TDP-43 proteinopathies [6] , given their shared TDP-43 IBs. Pathogenic TDP-43 was discovered in the urea fraction of the nervous tissues of FTLD-TDP and ALS patients [1] . The fraction contains aggregated forms, including high-molecular-weight aggregates and full-length and amino-terminus-truncated TDP-43, which are polyubiquitinated and hyperphosphorylated. The truncated TDP-43 that contains the carboxy-terminal fragment of TDP-43 and migrates as ~23–27 kDa after dephosphorylation were found only in the diseased tissues, but not in those of the age-matched controls. Recently, full-length TDP-43 species was also shown to present in aggregates associated with FTLD-TDP [7] . TDP-43 is normally located in the nucleus, but the IBs are predominantly cytoplasmic [1] , [8] . Although TDP-43 IBs resemble those found in many other neurodegenerative diseases with thioflavin-positive amyloid inclusions, TDP-43 IBs are not classified as amyloids as the pathologic amyloid staining results are not yet conclusive [6] , [9] . Amyloids are defined as proteins prone to aggregate into amyloid fibrils composed of specific cross-β structures [10] , which can be probed by ThT and Congo Red. Although amyloid fibrils in IBs are the pathologic hallmarks in many neurodegenerative diseases, many biochemical and animal studies have demonstrated that intermediate, spherical, amyloid oligomers are the major culprits to cause neurodegeneration [11] , [12] , [13] . Thus, a common disease mechanism associated with amyloid oligomers has been suggested among the neurodegenerative diseases [14] , [15] . Human TDP-43 is composed of 414 amino acids with two RNA recognition motifs (RRMs) and flexible regions in the N- and C termini ( Supplementary Fig. 1a ). TDP-43 has multiple functions in gene transcription and translations [3] , [16] . RRMs of TDP-43 bind to both single- and double-stranded TG-DNAs and UG-rich RNA [17] , and HIV trans-activation response element (TAR) DNA [18] . TDP-43 dimerization has been shown by size-exclusion chromatography (SEC) of the green fluorescent protein-tagged protein and from an examination of the structure of mouse RRM2 in complex with a single-stranded RNA [17] . The C-terminal region of TDP-43 is highly disordered [19] and contains a glycine-rich domain and a prion-like GQN sequence [16] . The aetiology of FTLD-TDP and ALS remains unclear with respect to loss-of-function and gain-of-toxicity effects supported by the literature. Deletion of TDP-43 is embryonically lethal, suggesting that dysregulation of RNA metabolism mediated through a TDP-43 defect probably contributes to the toxicity [20] . The TDP-43 mutant transgenic mice developed disease symptoms in the absence of cytoplasmic TDP-43 aggregates, which suggests that the loss-of-function of TDP-43 contributes to its pathogenesis [21] . On the other hand, overexpression of the full-length or N-terminus-truncated TDP-43 in yeast is toxic and forms cytoplasmic aggregates [22] . The rats injected with a viral TDP-43 construct have undergone neuronal apoptosis [23] , and TDP-43 transgenic mice partially recapitulate ALS and FTLD-TDP [24] , [25] . Despite the emerging biological studies on the pathogenic role of TDP-43, several studies have suggested that RRM1 (refs 26 , 27 ), RRM2 (ref. 28 ) and the glycine-rich domain [19] , [29] , [30] play roles in aggregation. However, detailed characterization of the full-length TDP-43 aggregates and the toxicity is still limited. Here, by various biochemical and biophysical methods, we discovered that full-length TDP-43 readily forms spherical oligomers that shared common epitopes with amyloid oligomers. The TDP-43 oligomers are conformational and functional distinct to native TDP-43 and are neurotoxic. Interestingly, the oligomers can convert amyloid-β (Aβ) to form Aβ oligomers rather than fibrils. We also provided evidence that these oligomers are present in the transgenic TDP-43 mice and FTLD-TDP patients. Our results suggest that TDP-43 oligomers are part of TDP-43 pathogenesis. Full-length TDP-43 readily forms aggregates To understand the mechanism of TDP-43 pathology, we first produced recombinant full-length human TDP-43 in Escherichia coli (TDP-43 with N-terminal His-Tag, molecular weight (MW) 47,145 Da, Supplementary Fig. 1b ). The purified TDP-43 was injected into an analytical SEC to analyse its assembly ( Fig. 1a ). We found >86% of TDP-43 was eluted in the void volume. Based on the MW standards, the species was larger than 440 kDa. We further injected the TDP-43 protein purified from HEK293 cells to SEC and analysed by slot blotting. The result also showed that TDP-43 was eluted in the void volume ( Fig. 1a and Supplementary Fig. 2 ), indicating that the majority of the recombinant full-length TDP-43 proteins from two different sources readily formed large aggregates. As TDP proteinopathies are characterized by IB formation and high MW aggregates were found in the recombinant full-length TDP-43, we suspected that TDP-43 may form oligomers resembling the amyloid oligomers in amyloidosis [31] . Therefore, we employed the conformation-dependent anti-amyloid oligomer-specific antibody, A11, generated against Aβ oligomer mimics to examine the TDP-43 oligomers [13] . A11 has been demonstrated to recognize common amyloid oligomers in various amyloidoses [13] . Here we examined the freshly purified TDP-43 and the void volume peak eluted from SEC designated as the oligomer fraction by dot blotting analysis ( Fig. 1b and Supplementary Fig. 3 ). Both TDP-43 samples, but not the corresponding buffers, were immunoreactive with A11. The oligomer fraction containing diluted TDP-43 exhibited weaker intensity. 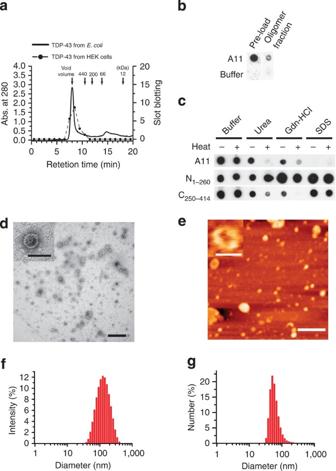Figure 1: Full-length TDP-43 forms amyloid-like oligomers. (a) Analytical SEC of full-length TDP-43 purified fromE. colimonitored by absorption at 280 nm (solid line) or human HEK293 cells quantified by slot blotting intensity (dashed line). The retention times of the MW standards are indicated. (b) Dot blotting of TDP-43 using anti-amyloid oligomer antibody, A11. Freshly purified TDP-43 before (pre-load TDP-43) and after SEC (the void volume, TDP-43 oligomers), and the buffers were immunostained with A11. (c) Freshly purified TDP-43 was dotted in buffer or buffers containing 9 M urea, 7.2 M GdnHCl, or 2% SDS, with or without heating at 90 °C for 1 h. Three replicates were generated and probed separately by A11 antibody, anti-N-terminal TDP-43 antibody (residues 1–260) and anti-C-terminal TDP-43 antibody (residues 250–414). (d) TEM and (e) AFM images of TDP-43 oligomers (scale bar, 500 nm) and zoomed-in images of a single oligomer are shown in the upper left (scale bar, 50 nm). (f,g) DLS analysis of the oligomer fraction of TDP-43 from SEC. Particle diameters are plotted against scattered light intensity (f) and particle number (g). Figure 1: Full-length TDP-43 forms amyloid-like oligomers. ( a ) Analytical SEC of full-length TDP-43 purified from E. coli monitored by absorption at 280 nm (solid line) or human HEK293 cells quantified by slot blotting intensity (dashed line). The retention times of the MW standards are indicated. ( b ) Dot blotting of TDP-43 using anti-amyloid oligomer antibody, A11. Freshly purified TDP-43 before (pre-load TDP-43) and after SEC (the void volume, TDP-43 oligomers), and the buffers were immunostained with A11. ( c ) Freshly purified TDP-43 was dotted in buffer or buffers containing 9 M urea, 7.2 M GdnHCl, or 2% SDS, with or without heating at 90 °C for 1 h. Three replicates were generated and probed separately by A11 antibody, anti-N-terminal TDP-43 antibody (residues 1–260) and anti-C-terminal TDP-43 antibody (residues 250–414). ( d ) TEM and ( e ) AFM images of TDP-43 oligomers (scale bar, 500 nm) and zoomed-in images of a single oligomer are shown in the upper left (scale bar, 50 nm). ( f , g ) DLS analysis of the oligomer fraction of TDP-43 from SEC. Particle diameters are plotted against scattered light intensity ( f ) and particle number ( g ). Full size image To confirm whether the recognition is conformation dependent, we used different denaturing methods to destruct TDP-43 oligomers and subjected them to dot blotting by A11 as well as anti-N-terminal and C-terminal TDP-43 antibodies ( Fig. 1c ). The protein was incubated in various buffers, namely, with or without 9 M urea, 7.2 M GdnHCl, or 2% SDS, and further treated at 90 °C for 1 h. For A11 detection, heating did not significantly alter the detection signal in the native buffer. However, the signals were weakened in the presence of high concentrations of urea or GdnHCl, and were nearly abolished by additional heat treatment. The signals were not detected in the presence of 2% SDS, regardless of heating. In contrast, the anti-N-terminal antibody recognized TDP-43 consistently across all conditions, confirming that equal amounts of proteins were dotted. The recognition by the anti-C-terminal antibody was diminished or completely lost when the samples were denatured in urea and heating or when the samples were denatured in GdnHCl, with or without heating. These findings indicate that the epitope recognized by the anti-C-terminal TDP-43 antibody is altered in these denaturing conditions. Taken together, our results showed that the recombinant full-length TDP-43 readily forms high MW species, which share a common epitope with amyloid oligomers. These species are highly stable under chemical denaturation but are SDS sensitive. Full-length TDP-43 forms heterogeneous spherical oligomers Next, we observed the morphology of the aggregates by transmission electron microscopy (TEM) ( Fig. 1d and Supplementary Fig. 4 ) and atomic force microscopy (AFM) ( Fig. 1e and Supplementary Fig. 5 ). TEM revealed heterogeneous spherical species with several spheroid-shaped and ring-shaped features, whereas AFM revealed mostly spheroids but very few ring-shaped structures ( Fig. 1e , inset). The particle size distribution was calculated based on TEM images. Majority of the spherical particles measured around 40–60 nm in diameter ( Supplementary Fig. 4c ). The ring-shaped oligomer examined by AFM was 6 nm in height ( Supplementary Fig. 5 ). In addition, dynamic light scattering (DLS) of the oligomer fraction eluted from the SEC also showed a heterogeneous distribution, with the particle size ranging from 40 to 400 nm in diameter ( Fig. 1f ). The largest population of these particles had a diameter of around 50 to 60 nm ( Fig. 1g ), which is consistent with the results from the TEM studies. Combining our imaging and size distribution findings, our results showed that full-length TDP-43 formed heterogeneous particles with spherical ultra-structures. The results are consistent with a previous report, suggesting wild-type TDP-43 and ALS-linked TDP-43 mutants formed oligomers [32] . We found that structurally and immunologically, these TDP-43 species closely resembled spherical amyloid oligomers that are widely considered neurotoxic in several neurodegenerative diseases [11] . TDP-43 oligomers are conformational and functional distinct To further examine the TDP-43 oligomers, we characterized the secondary structure content by far-ultraviolet circular dichroism (CD) ( Fig. 2a ). Two double minima were observed close to 210 and 222 nm, which probably represent α-helical structures. The spectrum was different from the short-form mouse TDP-43 (residues 101–265, denoted as TDP-43s in plots) comprising two RRMs with mostly β-strands in its crystal structure [17] . The fluorescence spectra resulting from the excitation of the intrinsic aromatic residues showed emission maxima at ~340 nm, indicating the tyrosinyl and tryptophanyl residues of TDP-43 were solvent exposed ( Supplementary Fig. 6 ). Furthermore, to detect the exposed hydrophobic protein surfaces, we employed an extrinsic fluorescence dye Bis-ANS that usually probes partially unfolded intermediates on protein folding [33] . We found the full-length TDP-43 reacted with Bis-ANS to a greater extent than the short-form TDP-43 ( Fig. 2b ), which further suggested that full-length TDP-43 oligomers possessed different hydrophobic-exposed surface area than the short-form TDP-43. 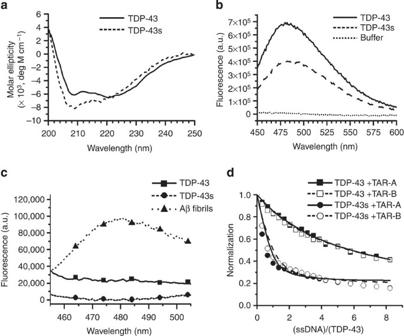Figure 2: Conformation, ThT fluorescence and DNA binding of TDP-43. (a) Far-ultraviolet CD spectra of full-length TDP-43 (solid line) and short-form TDP-43 (dashed line). The spectra from 250 to 190 nm are shown. (b) Bis-ANS fluorescence spectra of full-length TDP-43 (solid line) and short-form TDP-43 (dashed line). The buffer signal is shown (dotted line). (c) ThT binding of TDP-43 in comparison with Aβ fibrils. The ThT fluorescence emission spectra of full-length TDP-43 (▪, solid line), short-form TDP-43 (·, dashed line) and Aβ fibrils (▴, dotted line). Only Aβ fibrils showed ThT binding signal. (d) TAR DNA binding of TDP-43 monitored by fluorescence titration. Fullvlength (squares) and shortvform (circles) of TDP-43 were titrated with single-strand TAR DNA-A (solid symbols) and -B sites (empty symbols). The emission maxima of TDP-43 or TDP-43s at 350 nm were monitored while exciting at 280 nm. The data shown were normalized to the starting point and the lines shown are fit lines. Figure 2: Conformation, ThT fluorescence and DNA binding of TDP-43. ( a ) Far-ultraviolet CD spectra of full-length TDP-43 (solid line) and short-form TDP-43 (dashed line). The spectra from 250 to 190 nm are shown. ( b ) Bis-ANS fluorescence spectra of full-length TDP-43 (solid line) and short-form TDP-43 (dashed line). The buffer signal is shown (dotted line). ( c ) ThT binding of TDP-43 in comparison with Aβ fibrils. The ThT fluorescence emission spectra of full-length TDP-43 (▪, solid line), short-form TDP-43 (·, dashed line) and Aβ fibrils ( ▴ , dotted line). Only Aβ fibrils showed ThT binding signal. ( d ) TAR DNA binding of TDP-43 monitored by fluorescence titration. Fullvlength (squares) and shortvform (circles) of TDP-43 were titrated with single-strand TAR DNA-A (solid symbols) and -B sites (empty symbols). The emission maxima of TDP-43 or TDP-43s at 350 nm were monitored while exciting at 280 nm. The data shown were normalized to the starting point and the lines shown are fit lines. Full size image Moreover, we used the classic amyloid dye thioflavin T (ThT) to examine whether full-length TDP-43 binds to ThT. The spectra showed no fluorescence emission peak for either full-length or short-form TDP-43 resulting from ThT binding. By comparison, the Aβ fibrils at the same protein concentration, 1 μM, ( Fig. 2c ) showed strong fluorescence emission, consistent with the pathological examination result using thioflavin. Similarly, we examined TDP-43 oligomers binding with Congo Red ( Supplementary Fig. 7a ) and immunoreactivity with anti-fibrillar antibody OC ( Supplementary Fig. 7b ). The results were negative, contrary to the positive Aβ fibril controls. These results and the CD data show that TDP-43 oligomers are unlikely to adopt cross-β sheet structure. However, atomic level structural studies are needed for further characterization. Given that normal, functional TDP-43 binds to a specific nucleic acid sequence, we asked whether TDP-43 oligomers interfere with the DNA-binding capability. We first employed fluorescence titration to monitor protein conformational changes on DNA binding ( Fig. 2d ). TDP-43 oligomers were titrated with single-strand TAR DNA-A or -B sites and compared with the short-form TDP-43 that has been shown to bind these single-stranded DNAs (ssDNAs) in submicromolar affinity [17] . We found that both TAR DNA-A and -B sites quenched the short-form TDP-43 fluorescence in low ssDNA concentrations, whereas the level of quenching was significantly reduced in full-length TDP-43. The data fitted well with a single protein and ligand binding equation as described in Methods, indicating a 1:1 stoichiometry of TDP-43 and ssDNA. The dissociation constant, K d , obtained from the fits are 7.05±0.82, 6.27±0.68, 0.20±0.09 and 0.38±0.10 μM for full-length TDP-43 with TAR-A, full-length TDP-43 with TAR-B, short-form TDP-43 with TAR-A and short-form TDP-43 with TAR-B, respectively. The results showed that ssDNA binding for the short-form is >15-fold stronger than that for the full-length TDP-43 in which the TAR-A and -B sites have similar affinities to TDP-43. The finding indicate that RRMs of full-length TDP-43 oligomers either possess abnormal conformations with reduced DNA-binding capability or are hindered from DNA binding because of masking of the binding regions. The emission change that remained within the full-length TDP-43 could be attributed to the existence of a small population of TDP-43 monomers in the sample. Taken together, these results demonstrated that TDP-43 oligomers have different biophysical and biochemical properties from those of the short-form TDP-43, indicating their conformations are distinct. TDP-43 oligomers convert Aβ to amyloid oligomers Given the fact that recombinant full-length TDP-43 formed oligomers morphologically and immunologically similar to amyloid oligomers, we intended to test whether TDP-43 is able to influence Aβ fibrillization pathway through cross-seeding experiments. Aβ is a pathogenic protein in Alzheimer’s disease (AD), and its oligomerization and fibrillization are suggested to be causative factors of the disease. Structural conversion is a well-known phenomenon in prion pathology where the misfolded scrapie form PrP sc can convert native PrP c into scrapie form [34] . Seeding of amyloid fibrils with amyloid protein is often used to generate homogenous fibril species [35] or eliminate the nucleation step to form amyloid oligomers [36] , [37] . Recently, oligomer cross-seeding of Aβ and α-synuclein to induce toxic τ-oligomers was demonstrated [38] . Here we examined Aβ40 fibrillization by ThT assay in the absence and presence of TDP-43 oligomers, ranging from 0.4 to 4%. Interestingly, TDP-43 potently inhibited Aβ fibrillization in a dose-dependent manner ( Fig. 3a ). The presence of 4% TDP-43 totally suppressed Aβ fibrillization during our experimental time of ~180 h. We then performed photo-induced cross-linking (PICUP) to examine the transient Aβ species appeared in the starting time point. We found that Aβ alone formed primarily monomers, dimers, trimers and tetramers after cross-linking, whereas TDP-43 oligomer served to seed more higher MW Aβ species ( Fig. 3b ). Aβ pentamers were observed dose dependently on TDP-43 addition. Moreover, two larger assemblies, migrating at ~55 kDa and smearing from ~105 to >210 kDa, were observed. The TDP-43 oligomer seeds were also probed in the assay ( Supplementary Fig. 8 ). In addition to the SDS-irresistant TDP-43 monomers, a ~55-kDa species and some species causing a smear from ~80 to >210 kDa were found. Further analysis using TEM imaging showed that Aβ did not undergo fibril formation, but rather was transformed into spherical oligomers with a diameter of <10 nm in the presence of 4% TDP-43 oligomers, whereas Aβ alone still formed mature amyloid fibrils as expected ( Fig. 3c ). The TDP-43 oligomer seeds retained the diameter of >50 nm, which was larger than those of Aβ oligomers ( Supplementary Fig. 9 ). These results showed that TDP-43 oligomers can induce the Aβ oligomer formation, indicating again that TDP-43 shares common properties with amyloids. 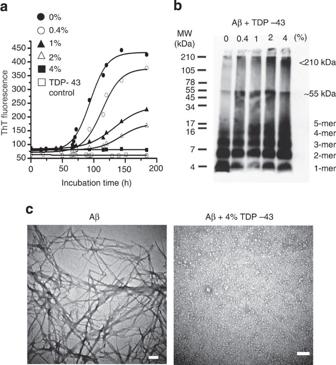Figure 3: Cross-seeding of TDP-43 to Aβ. (a) ThT assay of Aβ fibrillization without and with TDP-43 in concentrations ranging from 0.4% to 4%. Percentages of TDP-43 seeded in molar ratio are indicated. (b) Photo-induced cross-linking (PICUP) assay of Aβ without and with TDP-43 at time 0. The percentages of TDP-43 seeded in molar ratio are indicated. (c) TEM images of end-point products of Aβ without and with 4% TDP-43 (scale bar, 100 nm). Figure 3: Cross-seeding of TDP-43 to Aβ. ( a ) ThT assay of Aβ fibrillization without and with TDP-43 in concentrations ranging from 0.4% to 4%. Percentages of TDP-43 seeded in molar ratio are indicated. ( b ) Photo-induced cross-linking (PICUP) assay of Aβ without and with TDP-43 at time 0. The percentages of TDP-43 seeded in molar ratio are indicated. ( c ) TEM images of end-point products of Aβ without and with 4% TDP-43 (scale bar, 100 nm). Full size image TDP-43 oligomers induce neurite degeneration and toxicity With TDP-43 oligomers having biophysical properties similar to those of toxic amyloid oligomers, we investigated whether TDP-43 oligomers could cause neurotoxicity and neurite degeneration. We treated human neuroblastoma BE(2)-C cells with serially diluted TDP-43 sample containing predominantly oligomers, and examined the cytotoxic effect by MTT (3-(4,5-dimethylthiazol-2-yl)-2,5-diphenyltetrazolium bromide) and lactate dehydrogenase (LDH) assays ( Fig. 4 ). MTT assay results showed cytotoxicity with ~20% reduction in cell viability in the presence of 0.44 μM TDP-43 compared with the buffer controls ( Fig. 4a ). The poor solubility of recombinant TDP-43 made toxicity experiments with higher TDP-43 concentrations impossible. The LDH result also showed that 0.44 μM TDP-43 induced a significant amount of cell death ( Fig. 4b ). TDP-43 produced dose-dependent neurotoxicity in the primary cortical neurons of mice ( Fig. 4c ), where 0.6 μM of TDP-43 caused a ~20% reduction in cell viability. Immunohistochemistry of the treated cortical neurons of mice revealed that 0.6 μM TDP-43 induced shrinkage of neurites and reduced neuron density and numbers ( Fig. 4d ). To further test the neurotoxic effects of TDP-43 oligomers in vivo , we injected 2 μl of 2.2 μM TDP-43 to the hippocampal region of mice and examined the survival of neuronal cells by immunofluorescence staining. We found substantial loss of neuronal cells in the CA1 layer in TDP-43-injected mice ( Fig. 4e ), but not in the buffer-injected mice, as determined by the neuronal marker NeuN immunoreactivity and DAPI (4,6-diamidino-2-phenylindole) staining. The result showed that injection of recombinant full-length TDP-43 oligomers in the hippocampus can induce toxicity. 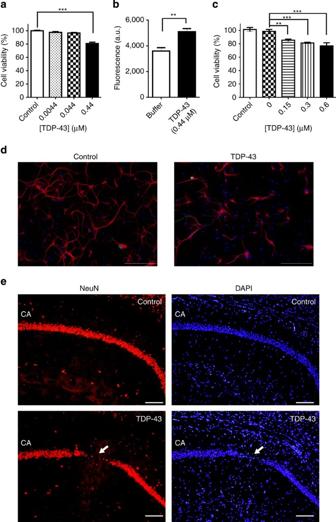Figure 4:TDP-43 oligomers induce neurite degeneration and are neurotoxicin vitroandin vivo. Cytotoxicity of TDP-43 to human BE(2)-C cells performed in (a) MTT and (b) LDH assays (n=3, mean±s.e.m.). (c) Cytotoxicity of TDP-43 to primary neuronal cultures using MTT assay. Cell viability in MTT assays is normalized against the buffer control (n=3, mean±s.d.). The statistics was analysed by one way-analysis of variance with Tukey’s post test foraandc, and two-tailed, unpaired Student’st-test forb(**P<0.01, ***P<0.001). (d) The immunocytochemistry of primary neurons treated with control or TDP-43, 0.44 μM. The samples were subjected to microtubule-associated protein-2 (MAP-2) immunostaining (red), glial fibrillary acidic protein (GFAP) immunostaining (green) and DAPI staining (blue). (e) Intrahippocampal TDP-43 injection showed neuronal loss in the CA regions of mouse hippocampus. Hippocampal injections (n=3 each) of the buffer control and TDP-43 were performed. Immunohistochemistry of the hippocampal regions with neuronal-specific marker NeuN and nuclear-specific dye DAPI are shown. The lesions are indicated by arrows (scale bar, 50 μm). Figure 4: TDP-43 oligomers induce neurite degeneration and are neurotoxic in vitro and in vivo . Cytotoxicity of TDP-43 to human BE(2)-C cells performed in ( a ) MTT and ( b ) LDH assays ( n =3, mean±s.e.m.). ( c ) Cytotoxicity of TDP-43 to primary neuronal cultures using MTT assay. Cell viability in MTT assays is normalized against the buffer control ( n =3, mean±s.d.). The statistics was analysed by one way-analysis of variance with Tukey’s post test for a and c , and two-tailed, unpaired Student’s t -test for b (** P <0.01, *** P <0.001). ( d ) The immunocytochemistry of primary neurons treated with control or TDP-43, 0.44 μM. The samples were subjected to microtubule-associated protein-2 (MAP-2) immunostaining (red), glial fibrillary acidic protein (GFAP) immunostaining (green) and DAPI staining (blue). ( e ) Intrahippocampal TDP-43 injection showed neuronal loss in the CA regions of mouse hippocampus. Hippocampal injections ( n =3 each) of the buffer control and TDP-43 were performed. Immunohistochemistry of the hippocampal regions with neuronal-specific marker NeuN and nuclear-specific dye DAPI are shown. The lesions are indicated by arrows (scale bar, 50 μm). Full size image Production of TDP-43 oligomer-specific antibody As the anti-amyloid oligomer antibody, A11, cross-reacted with different amyloids, to validate whether the TDP-43 oligomers are present in the disease, we generated a polyclonal antibody using the recombinant TDP-43 oligomers as immunogen in rabbit and named the polyclonal antibody TDP-O. We first examined the specificity of TDP-O antibody against the oligomeric conformation for the full-length TDP-43 by dot blotting coupled with different denaturing conditions as described in aforementioned method ( Fig. 5a ). TDP-O with 1:125,000 dilution was capable of recognizing full-length TDP-43 in the native buffer regardless of heating (90 °C, 1 h). The recognition disappeared when the samples were in the presence of 2% SDS with and without heating. Treating the full-length TDP-43 in either 7.2 M GdnHCl or 9 M urea at room temperature (RT) for more than 1 h did not weaken the recognition, indicating the protein was stable in high concentration of chemical denaturants. The signal was reduced when additional heating was performed, indicating TDP-O is a conformational-dependent antibody. The dot blotting result from TDP-O was qualitatively identical to that of A11 ( Fig. 1c ). 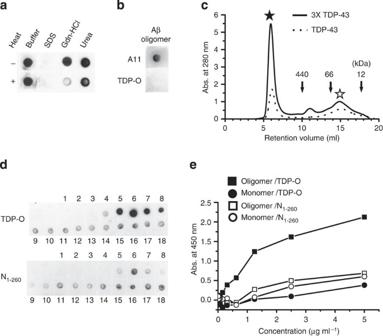Figure 5: TDP-O antibody recognizes TDP-43 oligomers specifically. (a) Freshly purified TDP-43 in native buffer or buffers containing 9 M urea, 7.2 M GdnHCl or 2% SDS, with or without heating at 90 °C for 1 h was subjected to dot blotting probed by the newly generated polyclonal antibody, TDP-O, using TDP-43 oligomers as immunogen. The immunoreactivity of TDP-43 conformation by TDP-O was similar to that by A11 as shown inFig. 1c. (b) Aβ oligomers were subjected to dot blotting probed by A11 and TDP-O antibodies. A11, but not TDP-O, was able to recognize Aβ oligomers. (c) TDP-43 with (solid line) and without (dotted line) threefold concentration were subjected to SEC. The elution volumes of TDP-43 oligomer (★), TDP-43 monomer (⋆) and the MW standards are indicated. (d) The 1-ml SEC fractions were collected and subjected to dot blotting by TDP-O (upper blot) and N1-260antibodies (lower blot). (e) The purified TDP-43 oligomers and monomers from SEC were characterized by ELISA. The TDP-43 samples were coated dose dependently onto the ELISA plates. The TDP-43 oligomers were probed by TDP-O (▪) and N1-260(□) antibodies, and TDP-43 monomers were probed by TDP-O (·) and N1-260(○) antibodies. TDP-O antibody possesses significant higher specificity against TDP-43 oligomers. Figure 5: TDP-O antibody recognizes TDP-43 oligomers specifically. ( a ) Freshly purified TDP-43 in native buffer or buffers containing 9 M urea, 7.2 M GdnHCl or 2% SDS, with or without heating at 90 °C for 1 h was subjected to dot blotting probed by the newly generated polyclonal antibody, TDP-O, using TDP-43 oligomers as immunogen. The immunoreactivity of TDP-43 conformation by TDP-O was similar to that by A11 as shown in Fig. 1c . ( b ) Aβ oligomers were subjected to dot blotting probed by A11 and TDP-O antibodies. A11, but not TDP-O, was able to recognize Aβ oligomers. ( c ) TDP-43 with (solid line) and without (dotted line) threefold concentration were subjected to SEC. The elution volumes of TDP-43 oligomer ( ★ ), TDP-43 monomer ( ⋆ ) and the MW standards are indicated. ( d ) The 1-ml SEC fractions were collected and subjected to dot blotting by TDP-O (upper blot) and N 1-260 antibodies (lower blot). ( e ) The purified TDP-43 oligomers and monomers from SEC were characterized by ELISA. The TDP-43 samples were coated dose dependently onto the ELISA plates. The TDP-43 oligomers were probed by TDP-O (▪) and N 1-260 (□) antibodies, and TDP-43 monomers were probed by TDP-O (·) and N 1-260 ( ○ ) antibodies. TDP-O antibody possesses significant higher specificity against TDP-43 oligomers. Full size image To test whether TDP-O is specific to TDP-43 rather than a common amyloid oligomer antibody such as A11, we examined the antibody specificity against Aβ oligomers by A11 and TDP-O ( Fig. 5b ). We found that TDP-O cannot recognize Aβ oligomers, demonstrating its specificity towards TDP-43 oligomers. Furthermore, we performed enzyme-linked immunosorbent assay (ELISA) to quantitatively characterize the recognition of TDP-43 oligomers and monomers with TDP-O in comparison with the TDP-43 antibody recognizing N-terminal residues 1–260 (N 1-260 ). To prepare the oligomer and monomer fractions of the full-length TDP-43, we injected either the full-length TDP-43 at ~1 μM or the three times more concentrated TDP-43 samples into SEC and collected 1 ml eluted fractions ( Fig. 5c ). We dotted the SEC fractions of the concentrated TDP-43 from fractions 1 to 18 and subjected them to dot blotting with TDP-O or N 1-260 antibodies ( Fig. 5d ). We found that TDP-O highly recognized fraction numbers 5–7 that corresponded to the TDP-43 oligomers eluted in the void volume. In contrast, N 1-260 showed higher recognitions in fractions 6 and 15–18, indicating that this antibody recognizes both oligomeric and monomeric TDP-43. Next, we quantified the TDP-43 oligomer specificity with TDP-O by ELISA where the N 1-260 antibody was used as control. After protein quantification by micro-BCA assay, the TDP-43 oligomer and monomer fractions were coated separately onto ELISA plate with serial dilutions. TDP-O and N 1-260 were applied and developed following standard ELISA protocol. The result showed that TDP-O antibody recognized TDP-43 oligomers (EC50 <0.5 μg ml −1 ) more robustly than TDP-43 monomer, whereas N 1-260 antibody recognized both TDP-43 oligomer and monomer similarly. Furthermore, to insure TDP-O recognizes the oligomeric rather than fibrillar form of TDP-43 as previously reported [28] , we dotted the β5 fibrils ( Supplementary Fig. 10b ) generated from the fifth β-strand within RRM2 domain of TDP-43 ( Supplementary Fig. 10a ). The result clearly showed that TDP-O recognizes only TDP-43 oligomers but not the β5 fibrils. Taken together, we demonstrated that our polyclonal TDP-O antibody specifically recognizes TDP-43 oligomeric conformation without cross-reacting with Aβ species. TDP-43 oligomers exist in transgenic mice brain To examine the presence of TDP-43 oligomers in vivo , we employed immunohistochemistry to stain the brain sections of wild-type mice and FTLD-TDP-43 transgenic mice at 6 and 12 month of age ( Fig. 6 ). This line of transgenic mice expressing full-length TDP-43 in the forebrain has been shown to recapitulate FTLD-TDP-like pathology [25] . The TDP-43 Tg mice were deficient in the learning/memory capabilities and motor functions with age. The brain sections were immunofluorescently stained with anti-TDP-43 and TDP-O, and counterstained with DAPI. In the wild-type mice, TDP-43 was found predominantly in the nucleus as expected. In the FTLD-TDP transgenic mice, TDP-43 deposited mainly in the cytosol and TDP-O signals were detected. Significant amount of TDP-43 and TDP-O signals colocalized and the cell with double-positive signals increased with age. The appearance and colocalization of the signals suggested that amyloid-like TDP-43 oligomers exist in the FTLD-TDP transgenic mice brain and increase with age. 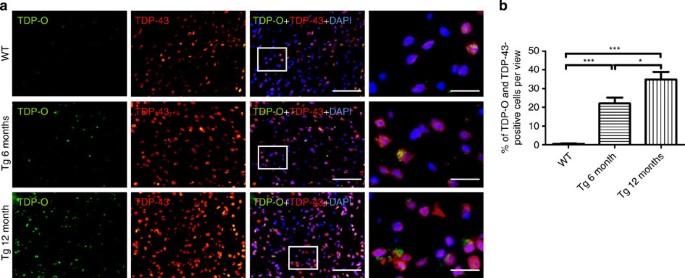Figure 6: TDP-43 oligomers are present and increase with age in transgenic mouse model of FTLD-TDP. (a) Immunofluorescent staining of human TDP-43 and TDP-43 oligomers in the brain slices of wild-type and 6- and 12-month-old TDP-43 Tg+/+ transgenic mice. Cells with anti-TDP oligomer staining (green), TDP-43 staining (red) and DAPI staining (blue) are shown (scale bar, 100 μm). Blocked area was presented at higher magnification in the last column (scale bar, 25 μm). (b) Quantified results showed that the ratio of cells with deposition of TDP-O and TDP-43 in cytosol were age dependent. (n=3 per group, random five views were calculated for each mouse, data are represented as mean±s.e.m.). The statistics was analysed by one way-analysis of variance with Tukey’s post test. *P<0.05, ***P<0.001). Figure 6: TDP-43 oligomers are present and increase with age in transgenic mouse model of FTLD-TDP. ( a ) Immunofluorescent staining of human TDP-43 and TDP-43 oligomers in the brain slices of wild-type and 6- and 12-month-old TDP-43 Tg+/+ transgenic mice. Cells with anti-TDP oligomer staining (green), TDP-43 staining (red) and DAPI staining (blue) are shown (scale bar, 100 μm). Blocked area was presented at higher magnification in the last column (scale bar, 25 μm). ( b ) Quantified results showed that the ratio of cells with deposition of TDP-O and TDP-43 in cytosol were age dependent. ( n =3 per group, random five views were calculated for each mouse, data are represented as mean±s.e.m.). The statistics was analysed by one way-analysis of variance with Tukey’s post test. * P <0.05, *** P <0.001). Full size image TDP-43 oligomers are present in brains of FTLD-TDP patients To evaluate the relevance of TDP-43 oligomers in human diseases, we examined whether TDP-43 oligomers are present in FTLD-TDP patients, the subgroup of FTLD patients with TDP-43 immunoreactive inclusions. We used the TDP-O antibody to immunostain hippocampal and frontal cortical sections of three cases of pathologically confirmed FTLD-TDP, three cases of age-matched non-dementic controls and three cases of pathologically confirmed AD without TDP-43 pathology as the ‘disease controls’. The TDP-O antibody identified various neuronal cytoplasmic inclusions ( Fig. 7a,c ) and dystrophic neurites ( Fig. 7a ) that appeared to be similar to the TDP-43 inclusions in FTLD-TDP patients. In some areas, neuronal cytoplasm was intensively stained in a granular pattern ( Fig. 7e ). In contrast, except the nonspecific reactivities from neuronal lipofuscin, TDP-O did not show significant immunoreactivities in sections of the control brains ( Fig. 7b,d,f ) and AD brains without TDP-43 pathology ( Supplementary Fig. 11 ). TDP-O antibody did not stain the nuclei in normal tissue, which is consistent with our biochemical observation that it does not recognize TDP-43 monomer normally present in the nuclei. In addition, to validate the morphology of TDP-43 recognized by TDP-O antibody, we performed immunoprecipitation (IP) by TDP-O with the control and diseased human hippocampus. The Triton soluble fractions of hippocampus were prepared and subjected to IP with cross-linked TDP-O antibody. The eluent was subjected to EM immunolabelled with N-terminal TDP-43 antibody (N 1-260 ) ( Fig. 8 ). We successfully observed rounded, spherical TDP-43 aggregates with a diameter of ~50 nm in the diseased sample but not in the control sample, and the species were recognized by N 1-260 antibody, indicating they are not N-terminal truncated. Overall, by using our TDP-O antibody, we demonstrated that TDP-43 oligomers exist in the brains of FTLD-TDP patients. 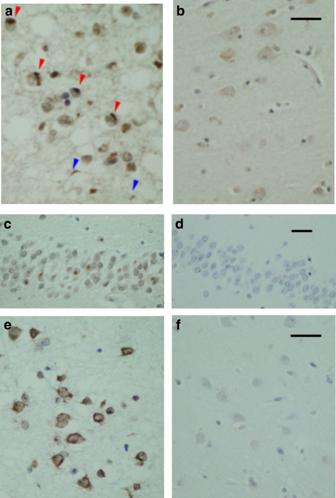Figure 7: TDP-43 oligomers are present in FTLD-TDP patients. A total of three FTLD-TDP cases, three neurologically and pathologically normal age-matched controls and three Alzheimer’s disease cases without TDP-43 inclusions (as ‘neurodegenerative disease controls’) were examined (seeSupplementary Fig. 11). Representative images are shown. (a,c,e) Immunohistochemical staining of TDP-43 in the hippocampal (c) and frontal cortical sections (a,e) of FTLD-TDP patients by the TDP-O antibody. TDP-O identified densely stained, ovoid or irregularly shaped but discreet cytoplasmic inclusions (red arrowhead), as well as comma-shaped profiles in the neuropil representing dystrophic neurites (blue arrowhead). In some cortical areas such as shown ine, neuronal cytoplasm showed coarse granular immunoreactivities. (b,d,f) TDP-O did not stain the brains of control subjects. TDP-O antibody, in contrast to antibodies for monomeric TDP-43, did not stain nuclei, demonstrating specificity toward misfolded TDP-43. Scale bars, 20 μm. Figure 7: TDP-43 oligomers are present in FTLD-TDP patients. A total of three FTLD-TDP cases, three neurologically and pathologically normal age-matched controls and three Alzheimer’s disease cases without TDP-43 inclusions (as ‘neurodegenerative disease controls’) were examined (see Supplementary Fig. 11 ). Representative images are shown. ( a , c , e ) Immunohistochemical staining of TDP-43 in the hippocampal ( c ) and frontal cortical sections ( a , e ) of FTLD-TDP patients by the TDP-O antibody. TDP-O identified densely stained, ovoid or irregularly shaped but discreet cytoplasmic inclusions (red arrowhead), as well as comma-shaped profiles in the neuropil representing dystrophic neurites (blue arrowhead). In some cortical areas such as shown in e , neuronal cytoplasm showed coarse granular immunoreactivities. ( b , d , f ) TDP-O did not stain the brains of control subjects. TDP-O antibody, in contrast to antibodies for monomeric TDP-43, did not stain nuclei, demonstrating specificity toward misfolded TDP-43. Scale bars, 20 μm. 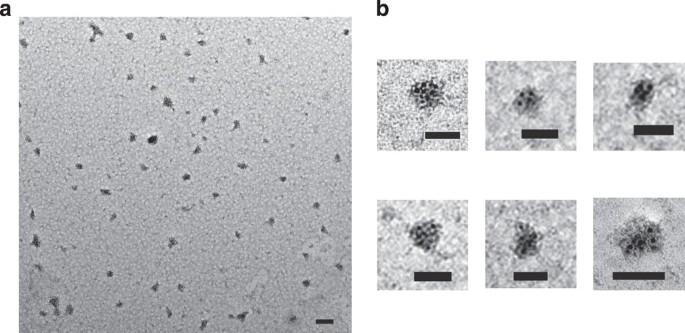Figure 8: Immunogold labelling of TDP-43 oligomers immunoprecipitated from the diseased hippocampus. The hippocampus of a FTLD-TDP patient was extracted and immunoprecipated by TDP-O antibody. The eluent was subjected to EM with immunogold labelling with the N-term TDP-43 antibody (scale bar, 50 nm). (a) TDP-43 oligomers in FTLD-TDP (scale bar, 100 nm) (b) zoom-in images of TDP-43 oligomers (scale bar, 50 nm). Full size image Figure 8: Immunogold labelling of TDP-43 oligomers immunoprecipitated from the diseased hippocampus. The hippocampus of a FTLD-TDP patient was extracted and immunoprecipated by TDP-O antibody. The eluent was subjected to EM with immunogold labelling with the N-term TDP-43 antibody (scale bar, 50 nm). ( a ) TDP-43 oligomers in FTLD-TDP (scale bar, 100 nm) ( b ) zoom-in images of TDP-43 oligomers (scale bar, 50 nm). Full size image Many neurodegenerative diseases, includingAD, Parkinson’s, and Huntington’s diseases are characterized by amyloidosis in which amyloid deposits are identified inside or outside the neurons [39] . Amyloid deposits comprising mature amyloid fibrils react with amyloid-specific dyes such as ThT, thioflavin S and Congo Red. However, amyloid oligomers, which are considered the major pathogenic culprits, react weakly with these dyes. The phenomenon has been discovered in many of those pathogenic proteins such as Aβ and τ in AD, α-synuclein in Parkinson’s disease and prions in prion diseases. Aβ in AD progressively aggregates into cross-β amyloid fibrils through a nucleation-dependent polymerization pathway [36] . The intermediate pre-fibrillar Aβ oligomers have been found to correlate best with cognitive impairment and synaptic dysfunction [11] . Various assemblies and morphologies of Aβ oligomer have been reported [40] in which pore-like oligomers have been suggested to form membrane permeable pores [31] and ion channels [41] . Our results demonstrated that TDP-43 oligomers are also heterogeneous. The dominant morphology resembles spherical oligomers found in Aβ and α-synuclein oligomers [42] . The fact that they are also neurotoxic suggests full-length TDP-43 may possess a pathogenic mechanism similar to other amyloid pathologies. However, considering that TDP-43 plays essential roles in normal physiology, other factors should also contribute to the pathogenesis. Filamentous ultra-structures have been observed in TDP-43 inclusions in FTLD-TDP and ALS brains [43] . Biochemical studies have shown that the recombinant full-length TDP-43 and ALS mutants are prone to aggregation [32] , and filamentous ultra-structure were observed with phosphorylated TDP-43 (ref. 44 ). Two core aggregation regions were found by synthetic peptides spanning the C terminus of TDP-43 (ref. 30 ). They are residues 311–320 within the disordered C-terminal region of TDP-43, which plays a more crucial role in nucleation, and 246–255 within the RRM2. The C-terminal peptide fragment (residues 287 to 322), and the third (residues 227–233) and fifth (residues 253–259) β-strands in RRM2 are also capable of forming ThT-negative, β-rich fibrils [19] , [28] . In addition, oxidative stress-induced disulphide bond formation via cysteine residues within and close to RRM2 and RRM1 affects TDP-43 oligomerization [27] , [45] . Whether the TDP-43 oligomers assemble via these regions is unknown, because the aggregated morphologies between our full-length oligomers and fibrils formed from peptides are distinct. However, those aggregation-prone regions are also possibly involved in oligomer formation. TDP-43 has been discovered in both sporadic and familial AD [46] , [47] , [48] , and our seeding results showed that TDP-43 oligomers can interact and influence Aβ fibrillization. The increased Aβ assembly in the presence of TDP-43 could result from a seeding effect that generates new Aβ assemblies such as Aβ*56 and larger aggregates or formation of cross-linked TDP-43 and Aβ complexes. The latter case may be more probable, as TDP-43 also migrated in similar MW regions. Whether TDP-43 and Aβ interact physiologically or play a role in the corresponding diseases is currently unknown, and it requires further investigation. Recently, prion-like propagation of TDP-43 itself has been shown in diseased brains [49] . Our study provided an evidence for the first time that TDP-43 oligomer can convert Aβ to amyloid oligomers, which suggests that TDP-43 has similar properties of amyloidogenic proteins, and the oligomers may play a role in AD. Overall, our results demonstrated that a possible pathologic mechanism of TDP-43 proteinopathies is linked to the generation of toxic amyloid oligomers. Our biochemical studies showed that the intrinsic protein properties of full-length TDP-43 readily allow it to form spherical and soluble amyloid oligomers with neurotoxicity in vitro and in vivo . The toxicity induced by extracellular TDP-43 treatment in our studies support prion-like spreading property of aggregated TDP-43 (ref. 49 ). Such TDP-43 oligomers exist in the FTLD-TDP patients as proven by our conformational-dependent TDP-43 antibody and confirmed by immunolabelling. Our result on the toxicity of the full-length TDP-43 is consistent with the studies showing that TDP-43 neurotoxicity in Caenorhabditis elegans is independent of caspase-3 cleavages [50] and elevation of TDP-43 expression in the forebrain of mice is sufficient to generate FTLD-TDP-like pathology, in which the TDP-43 generates large insoluble aggregation without much truncated species [25] . At this point, whether the truncated TDP-43 also forms amyloid oligomers and the exact role of such oligomers in the pathogenesis remain unknown. The pathogenesis, toxicity and amyloid oligomer-forming ability among full-length, truncated and modified TDP-43 should be further investigated. Materials The isolated human TDP-43 from HEK cells was a gift from OriGene Technologies, Inc. (Rockville, MD, USA). Based on the product description, TDP-43 was obtained from transiently transfected human HEK 293 cells with a TrueORF clone, RC210639. The recombinant TDP-43 possessed a C-terminal Myc-DDK tag. The overexpressed recombinant TDP-43 protein was purified using an anti-DDK affinity column. The short-form of TDP-43 (residues 101–285) [17] was a gift from Dr H.S. Yuan, Institute of Molecular Biology, Academia Sinica. Anti-N-terminal residues 1–260 TDP-43 antibody (denoted as N 1-260 ) for dot blotting and anti-TDP-43 antibody for immunohistochemistry were both purchased from Abcam (Cambridge, UK). Anti-C-terminal residues 350–414 TDP-43 antibody (denoted as C 350-414 ) was from Novus (Littleton, CO, USA) and anti-amyloid oligomer antibody A11 was from BioSource (Invitrogen, Carlsbad, CA, USA). Anti-DDK monoclonal antibody was from Origene Technologies, Inc. Aβ peptide was synthesized by peptide synthesis facility in the Genomics Research Center, Academia Sinica. Other chemicals were purchased either from Sigma Aldrich (St Louis, MO, USA) or Amresco (Solon, OH, USA). All cell culturing reagents were purchased from Gibco (Invitrogen), except for further indication. Purification of TDP-43 The N-terminal His-Tag TDP-43 was cloned from the plasmid pCMV-Taq2B containing the complementary DNA encoding full-length TDP-43, a gift from Dr P.H. Tu, Institute of Biomedical Sciences, Academia Sinica. The amplified product was double digested with Xho I/ Bam HI and subcloned into pET14b vector (Novagen, Merck KGaA, Darmstadt, Germany) to generate an N-terminal His-tag. The N-terminal His-tagged TDP-43 was transformed and overexpressed in E. coli strain Rosetta 2 (Novagen, Merck KGaA). The cells were harvested and lysed by a microfluidizer on ice in 30 mM Tris-HCl buffer, pH 8, containing 500 mM NaCl, 10% glycerol, 1 mM dithiothreitol, 2% RNase A, 2% DNase I and protease inhibitor cocktail (Complete, EDTA-free, Roche Applied Science, Mannheim, Germany). The lysate was centrifuged at 27,000 g , 4 °C. The supernatant was loaded onto Ni-NTA affinity column (GE Healthcare Bio-Sciences AB, Uppsala, Sweden) equilibrated in a buffer containing 30 mM Tris, pH 8, 500 mM NaCl, 1 mM dithiothreitol, 20 mM imidazole and 10% glycerol. Imidazole step gradients in the same running buffer were performed. TDP-43 was eluted at ~200 mM imidazole. Purified His-tagged TDP-43 protein was run on SDS–PAGE and identified by Coomassie blue staining ( Supplementary Fig. 1b ). The recombinant TDP-43 contained extra N-terminal residues MGSSHHHHHHSSGLVPRGSHMLE. The calculated molecular mass is 47,147 Da. The protein was further dialysed as indicated. Protein concentration was quantified after background subtraction by absorption at 280 nm with the extinction coefficient of 44,920 cm −1 M −1 according to the equation described by Pace et al . [51] For the short-form of TDP-43, the extinction coefficient of 15,470 cm −1 M −1 was used. Size-exclusion chromatography Superdex-200 10/300 GL analytical gel-filtration column (GE Healthcare Bio-Sciences AB) was standardized by MW markers, ferritin (440 kDa), β-amylase (200 kDa), BSA (66 kDa) and cytochrome C (12.4 kDa) in the running buffer containing 30 mM Tris, pH 7.4, 150 mM NaCl. The flow rate was 0.5 ml min −1 . A volume of 300 μl of the recombinant TDP-43 from E. coli filtered by 0.2 μm filter membrane was injected into the Superdex-200 column. One-millilitre fractions were collected automatically by a fraction collector. The preload sample and the oligomer fraction were collected and subjected to dot blotting probed by A11 (1:1,000), with different exposure times due to much diluted signal from the oligomer fraction. The oligomer fraction was characterized with DLS. A volume of 100 μl of TDP-43 obtained from HEK cells at 2 μM were also examined with the same procedure. The fractions were analysed by slot blotting. Slot blotting Fractions of the SEC of TDP-43 isolated from HEK293 cells were examined by slot blotting because of their low concentration. A 200-μl aliquot of every 1 ml fraction was loaded onto a Bio-Dot SF microfiltration apparatus (Bio-Rad, Hercules, CA, USA) equipped with an in-house vacuum system. Anti-DDK monoclonal antibody (OriGene Technologies, Inc., Rockville, MD, USA) was used as primary antibody for the detection. Intensity was quantified by Image J 1.42 (National Institutes of Health, MD, USA). Dot blotting Purified TDP-43 was diluted ten times into 10 mM Tris-HCl buffer, pH 8, with or without denaturants. Each sample in different conditions contains either no denaturant, 9 M urea, 7.2 M GdnHCl, or 2% SDS. The final TDP-43 concentration was 0.4 μM. The samples were either incubated for 1 h at the RT or 90 °C. The TDP-43 samples, 2 μl, were dotted onto nitrocellulose membranes and were subjected to dot blotting. Briefly, after blocking and washing with Tris-buffered saline containing 0.002% Tween 20 (TBST), the membranes were subjected to anti-N-terminal residues 1–260 TDP-43 antibody (1:2,000), Anti-C-terminal residues 350–414 TDP-43 antibody (1:2,000) and anti-amyloid oligomer antibody, A11, (1:1,000) in 5% milk with TBST followed by the corresponding horseradish peroxidase-conjugated secondary antibodies anti-rabbit or anti-mouse IgG (1:5,000; Millipore, Billerica, MA, USA). The membranes were developed with electrochemiluminescence reagent (Millipore). Transmission electron microscopy Freshly purified TDP-43 was dialysed into a buffer containing 10 mM Tris, pH 8, at 4 °C overnight. The sample was centrifuged at 17,000 g at 4 °C for 30 min to remove precipitates, and the supernatant was quantified and subjected to TEM imaging. The TDP-43 samples were placed on glow-discharged, 400-mesh Formvar carbon-coated copper grids (EMS Inc., Hatfield, PA, USA) for 5 min, rinsed and negatively stained with 2% uranyl acetate. The samples were examined with Tecnai G2 Spirit TWIN TEM (FEI, Hillsboro, OR, USA) or Hitachi H-7000 TEM (Hitachi Inc., Japan) with an accelerating voltage of 75 kV. Atomic force microscopy Freshly purified TDP-43 was dialysed into a buffer containing 10 mM Tris, pH 8, at 4 °C overnight. The sample was centrifuged at 17,000 g at 4 °C for 30 min to remove precipitates, and the supernatant was quantified and subjected to AFM imaging. A volume of 10 μl TDP-43 was dropped onto freshly sliced mica (Ted Pella, Redding, CA, USA) and incubated for 5 min for sample adhesion. The sample was washed by 1 ml ddH 2 O and gently removed from the top of the tilted mica. The sample was left to dry in the RT and subjected to AFM imaging (Nanonics, Jerusalem, Israel) using tapping mode. AFM tips, PPP-ZEILR (Nanosensors, Neuchatel, Switzerland) with a spring constant of 1.6 N m −1 and the tip radius <10 nm were employed for the experiment. Dynamic light scattering The eluted oligomer fraction from SEC was used for DLS. The sample was in a buffer containing 30 mM Tris, pH 7.4, and 150 mM NaCl. Data were obtained with a Zetasizer Nano ZS DLS instrument (Malvern Instruments, Worcestershire, UK) equipped with 50 mW later fibre. Appropriate parameters of viscosity and refractive index were set for each solution and the temperature was kept at 25 °C. Circular dichroism Freshly purified TDP-43 was dialysed into a buffer containing 10 mM Tris, pH 8, at 4 °C overnight. The sample was centrifuged at 17,000 g at 4 °C for 30 min to remove precipitates, and the supernatant was quantified and subjected to CD measurement. Far-ultraviolet CD spectra were measured in a circular quartz cell (Hellma, Forest Hills, NY, USA) by Jasco J-815 spectropolarimeter (Jasco Inc., Easton, MD, USA) with 1 mm path length at RT. The spectra were collected from 250 to 190 nm and corrected with buffer background. Intrinsic and Bis-ANS fluorescence spectroscopy Freshly purified TDP-43 was dialysed into a buffer containing 10 mM Tris, pH 8, at 4 °C overnight. The sample was centrifuged at 17,000 g at 4 °C for 30 min to remove precipitates and the supernatant was quantified. The intrinsic fluorescence of TDP-43, at 1.5 μM, was collected from 305 to 400 nm, while excitation at 280 or 295 nm. The Bis-ANS spectra of TDP-43, TDP-43s and buffer control were collected from 450 to 600 nm with excitation at 400 nm. The samples contain 0.8 μM TDP-43 and 5 μM Bis-ANS. All experiments were done at 25 °C with a circulating water bath using FluoroMax-3 spectrofluorometer (Horiba Jobin Yvon, Kyoto, Japan). Thioflavin T binding Freshly purified TDP-43 was dialysed into a buffer containing 10 mM Tris, pH 8, at 4 °C overnight. The sample was centrifuged at 17,000 g at at 4 °C for 30 min to remove precipitates and the supernatant was quantified. The TDP-43 sample and Aβ40 fibrils were used to detect ThT binding. The samples, 1 μM, were mixed with equimolar ThT and excited at 442 nm, and the emission spectra from 455 to 505 nm were collected. Aβ40 fibril stock, 25 μM, was prepared as previously described [52] . Briefly, synthetic Aβ was dissolved in 6 M GdnHCl and re-folded to 10 mM phosphate buffer, pH 7.4. Next, Aβ, 25 μM, was incubated at 25 °C in quiescence for more than 10 days. The mature fibrils were then diluted to 1 μM before the experiments. The spectra were subtracted from the buffer background. Congo Red spectroscopy Absorbance of dialysed TDP-43 and mature Aβ fibrils, 0.5 μM, was measured from 400 to 600 nm in the presence of f 10 μM Congo Red by an ultraviolet–visible spectrophotometer DU800 (Beckman Coulter, CA). Dot blotting by OC antibody The dialysed TDP-43 and Aβ fibrils (2 μl, 0.5 μM) were dotted onto nitrocellulose membranes and standard dot blot procedure was performed. OC antibody (Millipore, 1:10,000) and horseradishperoxidase-conjugated anti-rabbit IgG (1:10,000) were employed. Fluorescence titration for DNA binding Fluorescence titration was employed to monitor protein conformational changes on DNA binding. Freshly purified and dialysed full-length TDP-43 and short-form of TDP-43 (residues 101–285), at 1.5 μM, in 30 mM Tris-HCl, pH 8, were titrated with single strand TAR DNAs, including TAR DNA A-site (5′- CTTTTTGCCTGT -3′) and B-site (5′- TGGGTCTCTCTG -3′). The intrinsic protein fluorescence was excited at 280 nm to monitor the conformational change of TDP-43. The emission spectra were collected by FluoroMax-3 spectrofluorometer (Horiba Jobin Yvon, NJ, USA). The emission maxima at 350 nm for full-length or short-form TDP-43 were collected, subtracted with the DNA controls and corrected with the dilution factor. Then, the data were normalized to the starting intensity and further fitted to a single protein and ligand binding equation [53] : where γ is the fraction of the observed signal changes representing the bound protein fraction, P t is the total TDP-43 concentration, L t is the total ligand concentration, and K d is the dissociation constant. The data and fits are plotted against the ratio of DNA and TDP-43. Oligomer cross-seeding and ThT assay Aβ was prepared following our previous protocol [54] , [55] . Aβ40 was dissolved in buffer A (10 mM sodium phosphate, pH 7.4) containing 8 M GdnHCl, refolded and quantified using absorption at 280 nm ( ε =1,280 cm −1 M −1 ). The experimental samples containing 25 μM Aβ, 50 μM ThT and different concentrations of freshly dialysed TDP-43 ranging from 0 to 1 μM (0–4%) were prepared in 10 mM Tris-HCl, pH 8, and 150 mM NaCl. The samples were then incubated in a 96-well ELISA plate in quiescence, sealed with a transparent film and monitored by a microplate reader (SpectraMax M5, Molecule Devices, Sunnyvale, CA, USA) at 25 °C at various times. ThT emission was measured at 485 nm while excitation was measured at 442 nm. Photo-induced cross-linking The experiment was performed as described previously [56] . Briefly, we prepared the Aβ stock by a buffer containing 8 M urea and 10 mM sodium phosphate, pH 7.4, to facilitate running of SDS–PAGE. Aβ samples at 25 μM were prepared in a buffer containing 10 mM Tris-HCl, pH 8, and 150 mM NaCl with or without TDP-43 at different concentrations as indicated. The samples were immediately subjected to PICUP assay. A 90% Aβ solution was mixed with 5% each of 3 mM Ru(Bpy) and 20 mM APS. After mixing, samples were exposed to a blue-light LED in a closed chamber with a manual switch for 30 s. The cross-linking reaction was stopped by adding the SDS–PAGE sample buffer and the samples were run on 16% Tris-tricine SDS–PAGE. All actions were performed without delay. The gel was subjected to western blotting with anti-Aβ antibody 6E10 (Chemicon Inc., Billerica, MA) recognizing Aβ residues 1–17 and anti-N-terminal TDP-43 1–260 antibody. Cytotoxicity of TDP-43 using human neuroblastoma To perform cytotoxicity of TDP-43, MTT (3-[4,5-Dimethylthiazol-2-yl]-2,5-diphenyl-tetrazolium bromide) and LDH (Promega, Madison, WI, United States) assays were first employed using human neuroblastoma BE(2)-C cells (ATCC number CRL-2268). The cells were cultured in RPMI growth medium (Gibco) with 10% fetal bovine serum (Biological Industry) at 37 °C under 5% CO 2 and humidified atmosphere. A total of 60,000 cells per well was seeded in transparent 96-well ELISA plate (Corning, NY, USA) and incubated overnight. The cells were then washed and replaced by 40 μl of serum-free RPMI media followed by addition of 10 μl serially diluted TDP-43 samples with the dialysis buffer. The TDP-43 samples were freshly dialysed and centrifuged. The supernatant was employed and the dialysis buffer served as a buffer control. The cells were further incubated for 24 h and MTT assay was performed following the standard protocol. In brief, a volume of 7 μl of 5 mg ml −1 MTT was added in each well and cells were incubated for 3 h. Then, the media were discarded and dimethylsulphoxide was added to lyse the cells until the purple formazan crystals were fully dissolved. Absorbance at 570 and 690 nm were measured by an ELISA plate reader (SpectraMax M5, Molecule Devices) and the signals at 570 nm were subtracted from that of 690 nm. The data obtained from five replicas were averaged and corrected with the sample background without cells. The cell viability was shown after normalization of the data using the cell treated with buffer as 100%. LDH assay was performed following the manufacturer’s protocol. Briefly, a number of 20,000 cells was seeded in the growth medium and incubated for 24 h. The samples were treated as described in MTT assay. LDH substrate was mixed with the assay buffer and kept at RT. The cells were cooled to RT for 30 min before substrate addition. After 1 h of dark incubation, the substrate fluorescence was excited at 560 nm and emission at 590 nm was measured by the ELISA plate reader. The data were obtained from three replicas, averaged and corrected by the sample background without cells. The P -values of MTT and LDH assays were calculated using unpaired Student’s t -test. Cytotoxicity of TDP-43 using mouse primary cortical neurons The pregnant C57BL/6JNarl mice were purchased from National Laboratory Animal Center (NLAC, Taiwan) with the approval of the Institutional Animal Care and Use Committee (IACUC) at National Yang Ming University, Taipei, Taiwan. Primary cortical neuronal cultures were generated from embryonic day 19 mice and were seeded in 96-well plates (2 × 10 5 cells per well) with neurobasal medium (21103049, GIBCO, USA) containing 2 μM FdU. After growing 8 days in vitro , primary neuronal culture were treated with freshly dialysed soluble TDP-43 for 24 h, and then incubated with 0.5 mg ml −1 MTT for 3 h. The dialysis buffer was served as buffer control. MTT formazan crystals were then dissolved by equal volume of lysis buffer containing 10% SDS and 20 mM HCl overnight. The absorbance at wavelength 570 nm in each well was measured on an ELISA plate reader (TECAN, Switzerland). The data were obtained from three replicas, averaged and corrected by the sample background without cells. The P -values for MTT assay were calculated using unpaired Student’s t -test. Immunocytochemistry Primary neuron cells were cultured on 24-well plates with 12 mm glass coverslips (3 × 10 5 cells per well) and each well was coated with poly- D -lysine. Cells were treated with TDP-43 (0.6 μM) or buffer control for 24 h at 37 °C in a humidified atmosphere with 5% CO 2 and were fixed by 4% paraformaldehyde (PFA) for 20 min at RT. Then, the cells were washed with PBS 10 min for three times and blocked with blocking buffer (PBS containing 0.3% Triton X-100 and 10% fetal bovine serum) for 1 h at RT. After blocking, cells were first hybridized by the primary antibodies of microtubule-associated protein-2 (MAB378, Millipore, USA) and polyclonal rabbit anti-glial fibrillary acidic protein (Z0334, DAKO, Glostrup, Denmark) for 2 h at RT and then hybridized by the fluorescent dye-conjugated secondary antibodies of Texas-Red-conjugated goat anti-mouse IgG (AbD Serotec, UK) or fluorescein isothiocyanate-conjugated goat anti-rabbit IgG (Millipore) for 1 h at RT. Finally, cells were mounted by mounting gel containing DAPI (VECTASHIELD+DAPI, H-1200, Vector Lab.) and observed by Olympus fluorescence microscope (BX-61, Olympus, Tokyo, Japan). Intrahippocampal injection of TDP-43 Two-month-old male C57/BL6J mice were applied to intrahippocampal injection, which were purchased and bred in animal center of National Cheng Kung University (NCKU) following the guidelines of IACUC of NCKU. Animals were anaesthetized with isoflurane inhalation (1.2% in oxygen) via a nose tube. Each animal received bilateral intrahippocamal injection of recombinant full-length TDP-43. The stereotaxic coordinates were in relation to bregma as follows: anteroposterior, −2 mm; mediolateral, ±1 mm; dorsoventral, −2 mm. The injection needle slowly approached to the desired depth and 2 μl TDP-43, 2.2 μM, was injected using a stainless-steel syringe needle (33-gauge) connected to a microsyringe (Hamilton Company, NV, USA) at an injection rate of 1 μl min −1 . The needle was left in place for an additional 5 min to limit the diffusion of the injected TDP-43. Immunofluorescent staining of the mouse brains Twelve-month-old male wild-type mice, and 6- and 12-month-old TDP-43 Tg+/+ transgenic mice were adopt for immunofluorescent staining. All mice were also cared in animal center of NCKU following the guidelines of IACUC of NCKU. Two weeks after TDP-43 injection, the adult mice were deeply anaesthetized and perfused transcardially with 4% PFA/0.01 M PBS, pH 7.4. The brain was removed and then stored in 30% sucrose/4% PFA solution overnight. Ten-micrometre-thick sections were treated with a blocking solution containing 0.2% Triton X-100 and 5% normal donkey serum in 0.01 M PBS at RT for 1 h. For the experiments of intrahippocampal injection, the sections were incubated in mouse monoclonal anti-NeuN (1:300, Millipore, Temecula, CA) at 4 °C overnight and Alexa Fluor 555-conjugated donkey anti-mouse antibody (1:300, Chemicon, Temecula, CA) at RT for 1 h. The sections were then counterstained with DAPI and mounted with fluorescent mounting medium (DAKO). All sections were examined under an upright fluorescent microscope (BX51, Olympus). For the colocalization study in transgenic mice, the sections were incubated with anti-TDP-43 antibody (1:1,000, Abcam, ab104223), TDPO (1:1,000, LTK BioLaboratories, Taiwan), Alexa Fluor 488-conjugated goat anti-rabbit antibodies and the Alex Fluor 555-conjugated donkey anti-mouse antibodies (1:300, Invitrogen). The sections were then incubated with DAPI and coverslipped with fluorescent mounting medium (fluorescent mounting medium; DAKO). All sections were examined in a laser scanning confocal microscope (Nikon TE2000EPFS-C1-Si). TDP-43 oligomer-specific antibody production and characterization The purified full-length TDP-43 was dialysed into 10 mM Tris-HCl, pH 8.0, at 4 °C and concentrated to ~0.2 mg ml −1 to serve as immunogen. New Zealand white rabbits were immunized with the immunogen following the standard protocol for polyclonal antibody production (LTK BioLaboratories, Taiwan). Briefly, the immunogen was injected 0.5 ml into the rabbit at 2-week intervals. After 6 injections, the rabbit was killed and the blood serum was obtained for usage. For characterization of TDP-O by dot blotting and ELISA, full-length TDP-43 was subjected to SEC (Superdex-200 10/300 GL, GE Healthcare Bio-Sciences AB) in a buffer containing 30 mM Tris-HCl, pH 8.0, and 150 mM NaCl with a flow rate of 0.3 ml min −1 . One millilitre fractions were collected and subjected to dot blotting probed by TDP-O and N 1-260 antibodies. The TDP-43 oligomer and monomer fractions were further quantified by Micro BCA Protein Assay Kit (Thermo Scientific, Rockford, IL) and coated onto ELISA plate with serial dilution. ELISA following the standard protocol was performed. Briefly, the coated samples were incubated overnight at 4 °C, then blocked for 2 h at RT with 10% skim milk in TBST. The plates were washed and probed by TDP-O (1:12,500 in 3% skim milk in TBST) or anti-N-terminal residues 1–260 TDP-43 antibody (1:1,000 dilution in 3% skim milk in TBST) for 2 h at RT. After washing, the plates were subjected to anti-rabbit horseradish peroxidase-conjugated secondary antibodies (1:1,000; Merck Millipore, Billerica, MA, USA) for 2 h at RT, washed, then developed by 100 μl 3,3',5,5'-tetramethylbenzidine (Merck Millipore, Billerica, MA, USA). The reaction was stopped with 100 μl 250 mM HCl and the absorbance was read at 450 nm by SpectraMax M5 (Molecular Device). Generation of β5 fibrils β5 peptide within RRM2 domain of TDP-43 fragment was chemically synthesized (MDBio, Inc., USA). The peptide was solubilized by acetonitrile and diluted ten times with PBS buffer (pH 7.4) at 5 mg ml −1 . The supernatant was collected after centrifugation at 17,000 g for 30 min and filtered through a 0.2-μm filter membrane (Pall, USA). Next, the sample was incubated in quiescence at RT for 7 days. β5 fibrils were formed and the morphology was observed by TEM. The sample was subjected to dot blotting probed by TDP-O antibody following the aforementioned procedure. TDP-O staining of the brain tissues of FTLD-TDP patients Paraffin-embedded tissue sections were de-waxed with three washes of xylene. Tissues were then hydrated through an alcohol gradient, followed by a 5-min wash in 1 × TBS. Antigen recovery was performed using 10 mM sodium citrate (pH 6) by microwaving for 15 min at full power (1,500 W). Endogenous peroxidase activity was blocked by incubating the tissue in 3% hydrogen peroxide in 1 × TBS for 20 min, followed by a 5-min wash in 1 × TBS. Nonspecific binding was blocked by incubating the tissues in 10% normal goat serum (Invitrogen) for 1 h at ambient temperature. Primary antibody was diluted at 1:1,000 in antibody buffer (1 × TBS supplemented with 5% BSA and 0.5% Tween-20) and applied to the tissues overnight at 4 °C. Slides were washed three times in wash buffer (1 × TBS/0.5% Tween-20). Biotinylated secondary antibodies were applied at 1:500 dilution in antibody buffer for 1 h at ambient temperature. Tissue was washed three times in wash buffer, then incubated with Vectastain ABC peroxidase reagent (Vector Labs, PK-6100) for 30 min, followed by one wash in 1 × TBS. The tissues were then exposed to 3, 3′-diaminobenzidine (DAB) peroxidase substrate reagent (Vector Labs, SK-4100) for 2–10 min to achieve optimal staining. Tissues were counterstained with Mayers Hematoxylin Solution (Sigma Aldrich) and then dehydrated through an alcohol gradient followed by a xylene wash. Tissue slides were mounted using Permount (Sigma Aldrich). Post-mortem brain samples from three control, three FTLD-TDP and three AD patients were provided by the Alzheimer’s Disease Center at University of California Davis. The study was approved by the Institutional Review Board. Informed consent to share research tissue after death was obtained from all patients. IP and immunolabelling of TDP-43 oligomers in FTLD-TDP brain The frozen brain tissues of two control and one FTLD-TDP patient were lysed at ~0.05 g ml −1 with a lysis buffer containing 50 mM Tris, pH 7.4, 150 mM NaCl, 0.5% Triton X-100 and protease inhibitor cocktail (Calbiochem, Merck Millipore). The lysed samples were homogenized on ice by a tissue grinder (Wheaton, NJ, USA). After homogenization, the soluble fractions were collected after centrifugation at 17,000 g for 10 min at 4 °C and saved for IP analysis. Before tissue fractioning, crossed-linked TDP-O antibodies on the IP beads were prepared following the manufacturer’s procedure. Briefly, a total of 40 μg of TDP-O antibody was incubated with 10 μl each of protein A and G Mag Sepharose Xtra (GE Healthcare) in the binding buffer (50 mM Tris pH 7.5, 150 mM NaCl) at RT for 1 h. After antibody binding on the beads, cross-linking was performed by cross-link reagent (50 mM dimethyl pimelimidate dihydrochloride and 200 mM triethanolamine, pH 8.9) at RT for 1 h and the reaction was stopped by the addition of 100 mM ethanolamine, pH 8.9, at RT for 30 min. Next, the soluble fractions of hippocampus were incubated with the TDP-O antibody-cross-linked IP beads at RT for 1 h. The unbound species were removed by at least six washes with the binding buffer. The targeted protein was eluted by Gentle Ag/Ab Elution Buffer (Thermo), pH 6.6, and the eluent was saved for EM imaging and immunogold labelling. For immunogold labelling, 10 μl of eluent was placed on 400-mesh Formvar carbon-coated copper grids (EMS Inc., Hatfield, PA, USA) for 5 min, washed by PBS and then blocked by 1% BSA in PBS solution at RT for 1 h. After blocking, the grids were labelled by N 1-260 antibody (1:5,000, ab57105, Abcam) in 0.1% BSA containing PBS solution at RT for 1 h and washed by high-salt Tween buffer (50 mM Tris, pH 7.5, 500 mM NaCl and 0.1% Tween-20) and PBS. After washing, grids were incubated with 6 nm gold-conjugated secondary anti-mouse IgG antibody (1:40, Jackson ImmunoResearch) at RT for 1 h. The unbound antibody was removed by high-salt Tween and PBS washes. Next, the grids were fixed by 1% glutaraldehyde containing PBS at RT for 10 min and washed six times by double distilled H 2 O. Finally, the grids were rinsed, negatively stained with 2% uranyl acetate and subjected to TEM imaging with FEI Tecnai G2 F20 S-TWIN TEM. How to cite this article: Fang, Y.-S. et al . Full-length TDP-43 forms toxic amyloid oligomers that are present in frontotemporal lobar dementia-TDP patients. Nat. Commun. 5:4824 doi: 10.1038/ncomms5824 (2014).